Synthesis and physical properties of a ball-like three-dimensional π-conjugated molecule Curved π-conjugated molecules with closed and three-dimensional (3D) structures, such as fullerenes and carbon nanotubes, have been the subject of intensive research due to their potential applications in molecular electronics. However, basic molecular skeletons of 3D molecules are limited because of the lack of a rational and selective synthetic method by organic synthesis. Here we report the synthesis of a 3D π-conjugated molecule based on the platinum-mediated assembly of four molecules of a stannylated trisubstituted benzene derivative forming a hexanuclear platinum complex with an octahedral shape, from which reductive elimination of platinum gave the target molecule. As many supramolecular transition metal–ligand complexes with 3D cages and polyhedral structures have been synthesized by self-assembly of ligands and metals, the current assembly/reductive elimination strategy could provide a variety of new 3D π-conjugated molecules with different structures and topologies, which are challenging to obtain using conventional synthetic methods. After the discovery of fullerenes [1] and carbon nanotubes (CNTs) [2] , curved π-conjugated molecules with closed and three-dimensional (3D) structures have been the subject of intensive research. This is not only for their structural beauty but also their many potential applications in molecular electronics [3] , [4] . For example, C 60 and C 70 derivatives have been used as charge transport materials in organic photovoltaics [5] , [6] , and CNTs have demonstrated promise as nanowires or active components in electronic devices such as the field-effect transistor [7] . However, despite these developments, basic molecular skeletons of 3D molecules are limited. This is due to the lack of a rational synthetic method, with fullerenes and CNTs being prepared by physical methods such as laser vaporization or arc discharge of carbon and combustion of aromatic hydrocarbons. A solitary exception is the rational synthesis of C 60 by Scott et al . [8] , which was based on a flash vacuum pyrolysis technique. However, the application of this strategy to other 3D molecules has been hampered owing to the low generality, long synthetic steps, harsh reaction conditions and poor overall yields. Therefore, development of a general, bottom-up synthetic route to 3D π-conjugated molecules by organic synthesis is not only a significant challenge but also a pivotal contribution to materials science. Recently, two-dimensional (2D) hoop-shaped π-conjugated molecules, in particular cycloparaphenylenes (CPPs), the simplest structural unit of armchair CNTs, have captured significant interest [9] , and three groups including our own have developed new synthetic methods for producing them [10] , [11] , [12] , [13] , [14] , [15] , [16] , [17] . Our method relies on the formation of a square-shaped tetranuclear aryl platinum complex by the transmetallation of arylmetal species and a platinum dihalide ( Fig. 1a ) [12] , [18] , [19] , [20] . The process of the complex formation can be regarded as a covalent bonding version of the self-assembly of structurally related coordination complexes of palladium and platinum macrocycles with, for example 4,4′-bipyridyl, in supramolecular chemistry ( Fig. 1b ) [21] , [22] , [23] . Once the covalently bonded complex has been formed, reductive elimination of platinum affords the CPPs. 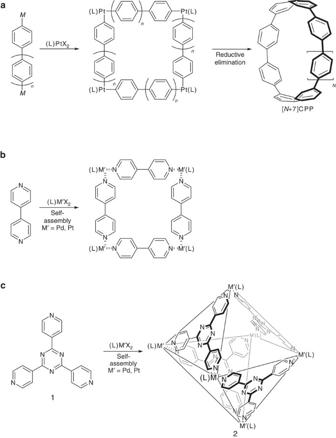Figure 1: Cycloparaphenylene and supramolecular transition metal–ligand complexes. (a) Synthetic route of cycloparaphenylenes (CPPs). (b) Self-assembly of metal–ligand interaction forming square metal complex. (c) Octahedral metal complex. M, metal; L, ligand. Figure 1: Cycloparaphenylene and supramolecular transition metal–ligand complexes. ( a ) Synthetic route of cycloparaphenylenes (CPPs). ( b ) Self-assembly of metal–ligand interaction forming square metal complex. ( c ) Octahedral metal complex. M, metal; L, ligand. Full size image As many supramolecular transition metal–ligand complexes with 3D cages and polyhedral structures have been previously reported [24] , [25] , [26] , [27] , it was envisioned that these complexes would be suitable precursors for 3D molecules. For example, Fujita [24] reported that trispyridyl ligand 1 and palladium(II) selectively and quantitatively formed octahedral, hexapalladium cage 2 by self-assembly involving a ligand–metal interaction. If a structurally related cage consisting solely of covalent bonds was to form, such a molecule would be a possible precursor of a 3D π-conjugated molecule. Here we report the synthesis of a 3D, spherical π-conjugated molecule, in which sp 2 -carbons of 1,3,5-trisubstituted and 1,4-disubstituted benzenes are covalently bonded forming a ball-like molecule. The synthesis involves the assembly of four molecules of tristannylated 1,3,5-benzene derivative and six platinum(II) species through 12-fold stannane–platinum transmetallation forming a hexanuclear platinum complex with octahedral shape, from which 6-fold reductive elimination of platinum gave the target molecule. The structure of the molecule is unambiguously determined by the single-crystal X-ray analysis. In addition, the optical and electrochemical properties and charge mobility of the molecule are reported. Synthesis of 3D molecule 3 The synthesis of 3D molecule 3 starting from commercially available tribromide 4a is summarized in Fig. 2 . Transmetallation of the bromide in 4a by BuLi, followed by the addition of trimethylstannyl chloride, gave 4b , which was treated with 3 equiv. of Pt(cod)Cl 2 (cod=1,5-cyclooctadiene) in 1,2-dichloroethane at 50 °C for 20 h, affording trisplatinated 4c in 75% yield (two steps). Subsequently, 4c was treated with an equimolar amount of 4b in 1,2-dichloroethane (1 mM) at 50 °C for 30 h. The white precipitate that was formed was collected by filtration and washed with 1,2-dichloroethane and toluene to afford 5d in 81% yield. The structure of 5d was characterized by 1 H and 13 C NMR spectroscopies. The formation of 5d is most likely to involve reversible C–Pt bond formation [18] , but the detail studies were hampered due to the low solubility of 5d . Treatment of 5d with bis(diphenylphosphino)ferrocene (dppf, 6 equiv.) gave 5e . After removal of cod and unreacted dppf, treatment of the reaction mixture with XeF 2 (6 equiv.) in toluene at 90 °C for 20 h gave 3 (refs 20 , 28 ), which was isolated by silica gel chromatography in 21% yield as a pale yellow solid. Using triphenylphosphine (6 equiv.) instead of XeF 2 also gave 3 , but in 19% yield. The use of bromine, however, which was employed in the synthesis of CPPs [12] , [18] , did not give the desired cyclic product at all. 3 was found to be soluble in many common solvents, including toluene, THF, CHCl 3 and CH 2 Cl 2 . 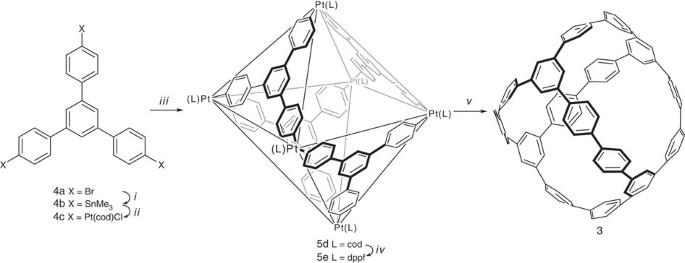Figure 2: Synthesis of 3. Reagents and conditions: (i) (1) BuLi (4.5 equiv.), THF, −78 °C, 1 h. (2) Me3SnCl (4.5 equiv.), −78 °C to room temperature, 6 h, 91%. (ii) Pt(cod)Cl2(3.0 equiv.), 1,2-dichloroethane, 50 °C, 20 h, 82%. (iii)4b(1.0 equiv.), 1,2-dichloroethane, 50 °C, 30 h, 81%. (iv) dppf (6.0 equiv.), CH2Cl2, rt, 19 h, 86%. (v) XeF2(6.0 equiv.), toluene, 90 °C, 20 h, 21%, or PPh3(6.0 equiv.), toluene, 90 °C, 20 h, 19%. cod, 1,5-cyclooctadiene; dppf, bis(diphenylphosphino)ferrocene. Figure 2: Synthesis of 3. Reagents and conditions: (i) (1) BuLi (4.5 equiv. ), THF, −78 °C, 1 h. (2) Me 3 SnCl (4.5 equiv. ), −78 °C to room temperature, 6 h, 91%. (ii) Pt(cod)Cl 2 (3.0 equiv. ), 1,2-dichloroethane, 50 °C, 20 h, 82%. (iii) 4b (1.0 equiv. ), 1,2-dichloroethane, 50 °C, 30 h, 81%. (iv) dppf (6.0 equiv. ), CH 2 Cl 2 , rt, 19 h, 86%. (v) XeF 2 (6.0 equiv. ), toluene, 90 °C, 20 h, 21%, or PPh 3 (6.0 equiv. ), toluene, 90 °C, 20 h, 19%. cod, 1,5-cyclooctadiene; dppf, bis(diphenylphosphino)ferrocene. Full size image The use of Pt complex was essential to obtain the octahedral complex. The use of Pd complex such as Pd(dppf)Cl 2 instead of the Pt complex resulted in a complex mixture because bis-aryl Pd complexes readily undergo reductive elimination and do not have sufficient lifetime to form the octahedral complex. The reductive elimination process was monitored by the 19 F and 31 P NMR spectroscopy ( Supplementary Figs S1 and S2 ). When XeF 2 (6 equiv.) was added to 5e in toluene-d 8 , the reaction mixture immediately turned orange. The 19 F NMR spectrum of the solution showed a singlet peak at −271.3 parts per million (p.p.m. ), suggesting the formation of single species. In the 31 P NMR spectrum, the singlet peak of 5e at 20.3 p.p.m. with a characteristic 195 Pt satellite ( 1 J PtP =1,784.3 Hz) completely disappeared and a new singlet peak at −2.9 p.p.m. with the satellite ( 1 J PtP =1,018.0 Hz) appeared. The large upfield shift and smaller 1 J PtP coupling constant of the product as compared with 5e suggested the formation of the corresponding (bis-aryl)Pt(IV)F 2 complex by the oxidation of 5e by XeF 2 (refs 28 , 29 , 30 ). After heating at 90 °C for 3 h, the 19 F NMR analysis indicated the complete disappearance of the signal at −271.3 p.p.m. and the appearance of a new singlet peak at −233.1 p.p.m. corresponding to Pt(dppf)F 2 together with several peaks from −290 to −236 p.p.m. The spectrum became simpler after 9 h of heating, and only the signal of Pt(dppf)F 2 was observed after 18 h. The same trend was observed in the 31 P NMR spectrum. The signal at −2.9 p.p.m. almost disappeared after 3 h with the formation of several new signals, and only a signal corresponding to Pt(dppf)F 2 was observed at 9.5 p.p.m. with the satellite ( 1 J PtP =3,542.3 Hz) after 18 h of heating. These observations suggest that the reductive elimination from the initially formed (bis-aryl)Pt(IV)F 2 to 3 did not proceed at the same time but rather in a stepwise manner. Characterization of 3 The product was first characterized in solution by NMR spectroscopy ( Supplementary Figs S3 and S4 ). In the 1 H NMR spectrum in CDCl 3 at 25 °C, 3 showed one singlet and two doublets in the aromatic region (7.41, 7.54 and 7.59 p.p.m. ), which is consistent with the highly symmetrical structure of 3 . This was also confirmed by the 13 C NMR spectrum, which showed six signals (125.5, 127.4, 128.3, 138.6, 139.5 and 141.9 p.p.m.). In the MALDI-TOF mass spectrum, a molecular ion peak was observed at m/z =1,212.4612, with an isotopic distribution pattern identical to the theoretical pattern ( Supplementary Fig. S5 ). The Raman spectrum of 3 in THF at room temperature shows a similar spectral pattern to that of CPPs [31] , but with approximately double the number of peaks present ( Supplementary Fig. S6 ). In addition to the peak derived from the paraphenylene unit, 3 showed the characteristic bands at 1,586, 1,329 and 1,231 cm −1 due to intra-ring C–C stretch, inter-ring C–C stretch and in-plane C–H bend, respectively, derived from the 1,3,5-trisubstituted benzene unit. 3D-structural information for 3 was first obtained by the density functional theory (DFT) calculations at the B3LYP/6-31G* level of theory. Six energy-minimized isomers with D 2 , S 4 , C 1 , C 2 , C 3 and T symmetries were calculated ( Fig. 3 ), among which the D 2 symmetric isomer was the most thermodynamically stable, followed by the S 4 symmetric isomer by 5.3 kJ mol −1 . The other isomers were found to be very high in energy (>16.0 kJ mol −1 ) compared with the D 2 isomer, suggesting that the contributions of these isomers to the ground state structure were negligible. As all isomers are rotational isomers with respect to the biphenyl units, the conversion among the isomers should occur spontaneously within the time frame of the NMR measurement. Indeed, the isomerization could not be frozen, even at low temperature, which was evident from the observation that the 1 H NMR signals of 3 did not split, even at −80 °C. 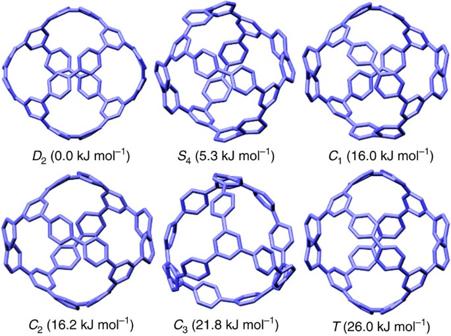Figure 3: Calculated structural isomers of 3. All molecular geometries were obtained by geometry optimization with DFT calculation at the B3LYP/6-31G* level. The energy values (kJ mol−1) beneath each isomer are the relative energy with respect to the lowest-lying isomer calculated at the corresponding level of DFT calculation. Blue represents carbon atoms. Hydrogen atoms are omitted for clarity. Figure 3: Calculated structural isomers of 3. All molecular geometries were obtained by geometry optimization with DFT calculation at the B3LYP/6-31G* level. The energy values (kJ mol −1 ) beneath each isomer are the relative energy with respect to the lowest-lying isomer calculated at the corresponding level of DFT calculation. Blue represents carbon atoms. Hydrogen atoms are omitted for clarity. Full size image The strain energy of the D 2 isomer was calculated to be 501 kJ mol −1 using a hypothetical homodesmotic reaction ( Supplementary Fig. S7 ). The strain energy of 3 is higher than that of [6]CPP (407 kJ mol −1 ), which is the smallest CPP that has been synthesized to date [20] , [32] , and even [5]CPP (491 kJ mol −1 ) [18] , [33] . In contrast, precursor 5 does not exhibit significant strain because the bond angle of cis -substituted platinum would be close to its ideal angle of 90°, although detailed structural analysis has so far proved unsuccessful. These results strongly suggest that the use of reductive elimination is an excellent strategy for synthesizing highly strained molecules. X-ray crystallographic analysis of 3 The structure of 3 was unambiguously determined by X-ray crystallographic analysis performed on a single crystal of 3 that was grown by vapor diffusion of n -hexane into a solution of 3 in CHCl 3 ( Supplementary Data 1 ). The crystal belongs to the tetragonal crystal system with a space group of P 2 1 c . As shown in the ORTEP drawing in Fig. 4a , 3 clearly exhibited a ball-shaped structure, with the inner void space occupied by highly disordered n -hexane molecules. The structure of 3 was found not to be a highly symmetrical circular shape but an elliptic form, the breadth of which was shown to be elongated along the c axis (15.28(3) Å) rather than the a - and b axes (12.54(9) Å), as estimated from the distance between the diagonal ipso carbon atoms. The conformation of 3 in the crystal did not have D 2 symmetry, which was calculated to be the most stable conformer, but instead possessed a pseudo S 4 symmetry, which was induced by the elongation of the c axis, as mentioned above. The bond lengths and bond angles of the crystal of 3 were in good agreement with those of the calculated S 4 structure, but the dihedral angle with respect to the two benzene units was slightly different. This apparent contradiction between the gas phase and crystalline structures is likely to be due to the effects of crystal packing forces and/or inclusion of solvent molecules. 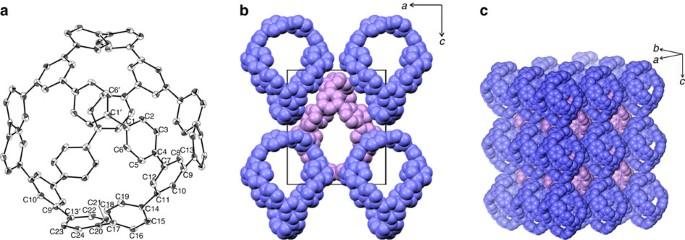Figure 4: Crystal structure of 3. (a) ORTEP drawing of3, showing the atom-numbering scheme. Asterisks indicate atoms generated by the symmetry operation. Thermal ellipsoids are shown at 50% probability. Hydrogen atoms and solvent atoms are omitted for clarity. Crystal data; tetragonal,P21c(#114):a=16.0885(6) Å,b=16.0885(6) Å,c=18.6558(8) Å,V=4828.9(3) Å3,Z=2,Rall=0.0665,wR2=0.1682, GOF=1.068. (b) Crystal packing of3. View downbaxis. (c) Space filling model in extended area. Carbon atoms are shown as blue or purple and layer structure (one layer in blue and another layers in purple) are presented in the figure. For clarity, hydrogen atoms and solvent molecules are omitted. Figure 4: Crystal structure of 3. ( a ) ORTEP drawing of 3 , showing the atom-numbering scheme. Asterisks indicate atoms generated by the symmetry operation. Thermal ellipsoids are shown at 50% probability. Hydrogen atoms and solvent atoms are omitted for clarity. Crystal data; tetragonal, P 2 1 c (#114): a =16.0885(6) Å, b =16.0885(6) Å, c =18.6558(8) Å, V =4828.9(3) Å 3 , Z =2, R all =0.0665, wR 2 =0.1682, GOF=1.068. ( b ) Crystal packing of 3 . View down b axis. ( c ) Space filling model in extended area. Carbon atoms are shown as blue or purple and layer structure (one layer in blue and another layers in purple) are presented in the figure. For clarity, hydrogen atoms and solvent molecules are omitted. Full size image Selected structural parameters of 3 obtained from the X-ray analysis and the theoretical calculations are summarized in Supplementary Table S1 . The bond lengths of the C ipso –C ipso bonds, namely C1–C1*, C4–C7, C9–C13, C11–C14 and C17–C20 were in the range of 1.46(4)–1.49(0) Å, the values of which are typical C ipso –C ipso bond lengths observed between two phenyl groups. The C–C bonds of the benzene rings were in the range of 1.37(7)–1.39(6) Å, and no significant bond alternation was observed. These results indicate that, despite extremely high strain of 3 , the benzenoid form was preserved in all of the benzene rings. This observation is in sharp contrast to the hexagons of fullerenes and small CPPs, where the benzenoid character is reduced owing to the presence of strain. The ipso carbon atoms were slightly pyramidalized, as indicated by the sum of three bond angles around them being <360° (357.4(2)–358.9(2)°). The bend angles as defined by the angle consisting of three ipso carbon atoms [33] , namely C1*–C1–C4, C1–C4–C7, C4–C7–C10, C12–C9–C13, C8–C11–C14, C11–C14–C17, C14–C17–C20, C17–C20–C13* and C20–C13*–C9* were 155.4(5)°, 158.1(1)°, 161.7(7)°, 161.7(7), 164.6(2)°, 161.3(1)°, 163.1(3)°, 163.4(7)° and 160.4(0)°, respectively. These observations suggest that the strain is more localized at the ipso carbons of the paraphenylene unit. The molecular arrangement of 3 in the crystal was found to be a body-centered quasi-cubic structure (a=b≠c), where each molecule of 3 in the unit cell center had eight nearest upside-down neighbors on the vertices of the unit cell, as shown in Fig. 4b and c . Interestingly, there is no π–π stacking contact of benzene units between adjacent molecules of 3 . Instead, weak off-set C–H/π interactions were observed between the central molecule and the vertex molecules, in which the C–H bonds lay perpendicular to the C atom of benzene, rather than pointing towards the center of the benzene rings ( Supplementary Fig. S8 ) [34] . The observed C–H…π bond distances (3.5–3.6 Å) were slightly longer than the sum of the van der Waals radius of sp 2 C (3.40 Å). This type of C–H…π interaction is observed in crystalline pentacene and is responsible for the large charge mobility in pentacene-based organic transistors [35] . Therefore, 3 might also serve as a new charge transport material in molecular electronics. Indeed, the flash-photolysis time-resolved microwave conductivity measurements [36] on the solid film of 3 with 7,7,8,8-tetracyanoquinodimethane gives a clear signature of photo-induced charge separation and the subsequent delocalization of positive charges on 3 , revealing its moderate hole mobility of 3.0 × 10 −3 cm 2 V −1 s −1 ( Supplementary Fig. S9 ). Physical properties of 3 The ultraviolet–vis spectrum of 3 in chloroform at room temperature shows an absorption maximum at 317 nm, with an absorption coefficient ε =29,000 M −1 cm −1 ( Supplementary Fig. S10 ). The time-dependent DFT calculations for the D 2 and S 4 isomers indicated that this absorption mainly consisted of four transitions for the D 2 isomer and three transitions for the S 4 isomer, but that the HOMO→LUMO transition was symmetry-forbidden for both isomers ( Supplementary Table S2 ). In the fluorescence spectra, a blue fluorescence was observed with λ em =426 nm in THF. The Stokes shift was significantly high, probably due to large structural relaxation from the Franck–Condon state [37] . The fluorescence quantum yield ( Φ F ) was determined to be 0.44, using 9,10-dicyanoanthracene as a standard. The fluorescence decay of 3 followed first-order kinetics with a lifetime ( τ )=2.1 ns, as measured by the single-photon counting method. The radiation decay rate constant ( k r ) was determined to be 2.1 × 10 8 s −1 from the equation k r = Φ F / τ . The electrochemical properties of 3 were studied using differential pulse voltammetry (DPV) in a 0.1 M solution of Bu 4 NPF 6 in 1,1,2,2-tetrachloroethane as a supporting electrolyte ( Supplementary Fig. S11 ). A single oxidation peak was observed, with an oxidation potential of +1.06 V versus ferrocene/ferrocenium couple (Fc/Fc + ); however, no reduction was observed under the given solvent window. A ball-like 3D π-conjugated molecule 3 was successfully synthesized and characterized. The key steps of the synthesis are the platinum-mediated assembly of π-units by transmetallation and subsequent reductive elimination of the platinum. The assembly process by which the hexanuclear platinum complex 5 was formed mimics the self-assembly of metal and ligands that form structurally related cage-like coordination complexes ( Fig. 1c ). Furthermore, despite the high strain of 3 , reductive elimination of platinum from 5 proceeded with reasonable yield. As many metal–organic frameworks with 3D structures are already known and can easily be prepared, the assembly/reductive elimination strategy described here would provide a variety of new 3D π-conjugated molecules with different structures and topologies, which are challenging to obtain using conventional synthetic methods. In view of the diverse range of possible functions of π-conjugated molecules, the current method has the potential to open up a new era of 3D π-conjugated molecules. Interestingly, as the structure of 3 is topologically identical to a Reuleaux triangle, the extension of this synthetic strategy should make it possible to synthesize molecules with Klein’s quartic curve structure [38] , a 3D version of a Möbius strip [39] . While this work was ongoing, Matsui et al . [40] reported on the synthesis of a π-conjugated 3D molecule that possessed a simpler bicyclic structure than 3 , which is tricyclic, using a modification of the strategy they developed for CPP synthesis. However, the synthesis required long reaction steps and the final product was only obtained in a low overall yield. Furthermore, it is likely that extension of the method to the synthesis of a structurally diverse array of 3D molecules would be challenging. General All reaction conditions dealing with air- and moisture-sensitive compounds were carried out in a dry reaction vessel under a nitrogen atmosphere. 1 H (400 MHz) and 13 C NMR (100 MHz) spectra were measured for a CDCl 3 or (CDCl 2 ) 2 solution of a sample and are reported in p.p.m. (δ) from internal tetramethylsilane or residual solvent peak. 19 F NMR spectra were measured at 376 MHz and are reported in δ from external C 6 F 6 (–162.9 p.p.m. ), which was separately calibrated from CCl 3 F (0.0 p.p.m.). 31 P NMR spectra were measured at 162 MHz and are reported from external 85% H 3 PO 4 aqueous solution. Infra-red spectrum (absorption) was reported in cm −1 . Electrospray ionization time-of-flight mass spectrum (ESI-TOF MS) was recorded under the positive mode with samples dissolved in a CH 2 Cl 2 /isopropanol solution. Matrix-assisted laser-desorption ionization time-of-flight mass spectrum (MALDI-TOF MS) was obtained on a spectrometer under the positive reflection mode with 20 kV acceleration voltage. Samples were prepared by mixing a 1:1 ratio of sample (1 mg ml −1 ) and dithranol (1 mg ml −1 ) solutions in THF. Ultraviolet–vis and fluorescence spectra were measured in CHCl 3 and THF at room temperature, respectively. DPV was performed with a Pt electrode of a sample solution (1 mM) in 0.1 M Bu 4 NPF 6 solution of 1,1,2,2-tetrachloroethane at room temperature under a nitrogen atmosphere. The scan rate with 20 mV s −1 was employed. After the measurement, ferrocene was added to the mixture and the potential was calibrated with respect to the Fc/Fc + . Materials Unless otherwise noted, commercially available materials were used without purification. Dichloromethane was distilled successively from P 2 O 5 and K 2 CO 3 and stored over molecular sieves. Toluene was distilled from CaH 2 and stored over molecular sieves. Pt(cod)Cl 2 (ref. 41 ), dppf (ref. 42 ), 1,3,5-tris( p -bromophenyl)benzene 4a (ref. 43 ) are commercially available and were easily synthesized as reported. 1 H NMR and 13 C NMR spectra are provided for all new compounds (see Supplementary Figs S12–S17 ). Synthesis of 4b To a solution of 4a (5.43 g, 10 mmol) in THF (75 ml) BuLi (32 ml, 1.41 M in hexane, 45 mmol) was slowly added by using a syringe at –78 °C. After stirring for 1 h at this temperature, a solution of trimethylstannyl chloride (8.96 g, 45 mmol) in THF (10 ml) was slowly added through a cannula at −78 °C and the resulting mixture was slowly warmed to room temperature over 3 h. After stirring for 3 h at this temperature, the reaction mixture was quenched with saturated aqueous NH 4 Cl solution and was extracted with ethyl acetate. The combined organic layer was washed with brine, dried over MgSO 4 , filtered and concentrated under reduced pressure to give a crude mixture. The residue was purified by passing neutral alumina with hexane as an eluent to give the title compound (7.22 g, 91%) as a white solid. 1 H NMR (CDCl 3 , 400 MHz) 0.34 (s, 27H, J Sn–H =54.0 Hz, SnMe 3 ), 7.62 (d, J =7.6 Hz, 6H, –ArH), 7.66 (d, J =7.2 Hz, 6H, –ArH), 7.77 (s, 3H, –ArH); 13 C NMR (CDCl 3 , 100 MHz) –9.50 ( J Sn–C =341.5 Hz), 125.18, 126.92, 136.35, 141.04, 141.50, 142.36; HRMS (FAB) m / z : calcd for C 33 H 42 Sn 3 (M) + , 798.0352; found 798.0285; IR (KBr) 798, 990, 1,265 1,420, 1,465, 1,571, 2,900, 3,002; mp 191.0–193.5 °C. Synthesis of 4c Pt(cod)Cl 2 (2.24 g, 6.0 mmol) and 4b (1.59 g, 2.0 mmol) were dissolved in 1,2-dichloroethane (1,200 ml) and the mixture was heated at 50 °C for 20 h under a nitrogen atmosphere. The solvent was removed under reduced pressure and the residue was washed with toluene to give a crude mixture. The residue was purified by passing over a short neutral alumina plug with CH 2 Cl 2 as an eluent to give the title compound (2.16 g, 82%) as a white solid. 1 H NMR (CDCl 3 , 400 MHz) 2.15–2.84 (m, 24H, cod), 4.65 (s, J Pt–C =68.5 Hz, 6H, cod), 5.81 (s, 6H, cod), 7.27–7.36 (m, 3H, –ArH), 7.36–7.49 (m, 6H, –ArH), 7.61–7.76 (m, 6H, –ArH); 13 C NMR (CDCl 3 , 100 MHz) 27.91, 32.13, 87.44 ( J CPt =201.3), 115.70, 124.30, 124.66, 127.11, 127.23, 128.71, 134.21, 137.28, 141.39, 141.84, 142.21, 143.43; HRMS (ESI-TOF) m / z : calcd for C 48 H 55 Cl 3 N 1 Pt 3 (M-NH 4 ) + , 1,337.2320; found 1,337.2402; IR (KBr) 772, 890, 986, 1,215, 1,460, 1,536, 2,221, 2,765, 2,980. Synthesis of 5d The solution of 4b (0.40 g, 0.5 mmol) and 4c (0.66 g, 0.5 mmol) in 1,2-dichloroethane (1,500 ml) was heated at 50 °C for 30 h under a nitrogen atmosphere, forming a white precipitate. The solvent was removed under reduced pressure and the residue was washed with 1,2-dichloroethane/toluene (1/1) to give the title compound (0.61 g, 81%) as a white solid. 1 H NMR (C 2 D 2 Cl 4 , 400 MHz) 2.17–2.65 (brs, 48H, cod), 4.84–5.27 (brs, 24H, cod), 7.18–7.23 (m, 24H, –ArH), 7.24–7.32 (m, 36H, –ArH); 13 C NMR (C 2 D 2 Cl 4 , 100 MHz) 30.48, 104.03, 126.83, 128.82, 130.05, 134.37, 135.55, 156.22; IR (KBr) 789, 988, 1,020, 1,088, 1,465, 1,568, 2,360, 2,868, 2,996. Synthesis of 3 A suspension of 5d (0.30 g, 0.1 mmol) and dppf (0.33 g, 0.6 mmol) in CH 2 Cl 2 (300 ml) was stirred at room temperature for 19 h under a nitrogen atmosphere. The solvent was removed under reduced pressure and the residue was washed with ethyl acetate to give 5e (0.49 g, 86%) as an orange solid. The suspension of 5e (0.49 g, 0.086 mmol) and XeF 2 (87.4 mg, 0.52 mmol) in toluene (86 ml) was heated at 90 °C for 20 h under a nitrogen atmosphere. The resulting suspension was filtered and the filtrate was concentrated under reduced pressure to give a crude mixture. The residue was purified by silica gel chromatography (hexane/CH 2 Cl 2 =4/1 to 1/1) to give 3 (21.9 mg, 21%) as a pale yellow solid. 1 H NMR (CDCl 3 , 400 MHz) 7.41 (d, 24H, J =8.0 Hz, –ArH), 7.54 (s, 12H, –ArH), 7.59 (d, 24H, J =8.0 Hz, –ArH); 13 C NMR (CDCl 3 , 100 MHz) 125.45, 127.36, 128.26, 138.55, 139.52, 141.89; HRMS (MALDI-TOF) m/z : calcd for C 96 H 60 [M] + : 1,212.4612; found 1,212.4690. Alternative synthesis of 3 A suspension of 5d (30.3 mg, 10 μmol) and dppf (33.3 g, 60 μmol) in CH 2 Cl 2 (30 ml) was stirred at room temperature for 19 h under a nitrogen atmosphere. The solvent was removed under reduced pressure and the residue was washed with ethyl acetate to give 5e (48.0 mg, 84%) as an orange solid. The suspension of 5e (48.0 mg, 8.4 μmol) and PPh 3 (26.4 mg, 101 μmol) in toluene (8.4 ml) was heated at 90 °C for 20 h under a nitrogen atmosphere. The resulting suspension was filtered off and the filtrate was concentrated under reduced pressure to give a crude mixture. The residue was purified by silica gel chromatography (hexane/CH 2 Cl 2 =4/1 to 1/1) to give 3 (1.9 mg, 19%) as a pale yellow solid. NMR monitoring of the reductive elimination of 5e To a solution of 5e (6.4 mg, 1.12 μmol) in toluene-d 8 (0.5 ml) in a NMR tube XeF 2 (67 μl, 0.1 M in toluene-d 8 , 6.72 μmol) was added at room temperature. The 19 F and 31 P NMR analyses showed the quantitative conversion from 5e ( 31 P NMR; 20.3 p.p.m., 1 J PtP =1,784.3 Hz) to the Pt(IV) difluoride complex ( 19 F NMR; −271.3 p.p.m., 31 P NMR; −2.9 p.p.m., 1 J PtP =1,018.0 Hz). The NMR tube was sealed and was heated at 90 °C. The progress of the reaction was monitored by 19 F and 31 P NMR spectrometry after 3, 9 and 18 h. The disappearance of 5e and the formation of several species were observed at 3 and 9 h and the reaction eventually gave Pt(dppf)F 2 ( 19 F NMR; 233.1 p.p.m., 31 P NMR; 9.5 p.p.m., 1 J PtP =3542.3 Hz) as an exclusive product. Computational study DFT calculations were carried out by using the Gaussian 09 program package [44] . The DFT method with the B3LYP hybrid functional [45] , [46] and the 6-31G(d) basis set [47] was employed. Geometry optimizations were performed under the constraint of D 2 , S 4 , C 1 , C 2 , C 3 or T symmetries. Normal coordinate analysis at the same level of theory was performed, and the number of imaginary frequencies was 0 for all structures. See Supplementary Figs S18 and S19 and Supplementary Tables S3 and S4 . X-ray crystallography Single-crystal X-ray diffraction experiments were carried out with a large cylindrical imaging plate camera [48] at SPring-8 beam line BL02B1 (Hyogo, Japan). Crystal data are summarized in Supplementary Table S5 . The structures were solved by the direct methods with SIR2004 (ref. 49 ) and refined by the full-matrix least-squares techniques against F 2 (SHELXL-97) [50] . The intensities were corrected for Lorentz and polarization effects. The non-hydrogen atoms were refined anisotropically. Hydrogen atoms were placed using AFIX instructions. All calculations were performed by using Crystal Structure 4.0 or Yadokari-XG 2011. Charge carrier mobility in 3 Charge carrier mobility in 3 was measured by the flash-photolysis time-resolved microwave (FP-TRMC) technique [36] , [51] . 3 (5 mg, 2.5 wt%) and 7,7,8,8-tetracyanoquinodimethane (5 mg, 2.5 wt%) were added to 200 mg of toluene solution including 5 wt% of poly(methyl methacrylate). The mixture was heated at 80 °C, casted onto a quartz substrate and dried at room temperature. The nanosecond laser pulses from an Nd: YAG laser (third harmonic generation, THG (355 nm) from Spectra Physics, INDI-HG, FWHM 4 ns) was used as excitation source. The excitation density was 4.6 × 10 15 photons cm −2 . The resonant frequency and the microwave power were set at ~9.1 GHz and 3 mW, respectively. The TRMC signal from a diode was recorded on a digital oscilloscope (Tektronix, TDS 3032B). The transient photoconductivity (Δσ) of the samples is related to the reflected microwave power (Δ P r / P r ) and sum of the mobilities of charge carriers via: where A , e , , N and ∑μ are the sensitivity factor, elementary charge of electron, photo carrier generation yield (quantum efficiency), the number of absorbed photons per unit volume, and sum of mobilities for negative and positive carriers, respectively. The value of was determined by transient absorption spectroscopy measurement. Details of the experimental setup are described elsewhere [36] . Time-dependent absorption spectral changes were monitored by Hamamatsu C7700 streak camera via a Hamamatsu C5094 spectrometer upon direct excitation of the identical solid-state films used for TRMC measurements using a third harmonic generation ( λ =355 nm, 50 mJ pulse −1 cm −2 ) from the Nd: YAG laser. To correct a 2D time–wavelength correlation data of the transient absorption, the streak scope images were averaged over 2,500 images via a high-speed camera (Hamamatsu C4742-95). Accession codes: The X-ray crystallographic coordinates for structures reported in this Article have been deposited at the Cambridge Crystallographic Data Centre (CCDC) under deposition numbers CCDC 924350. These data can be obtained free of charge from The Cambridge Crystallographic Data Centre via www.ccdc.cam.ac.uk/data_request/cif . How to cite this article: Kayahara, E. et al . Synthesis and physical properties of a ball-like three-dimensional π-conjugated molecule. Nat. Commun. 4:2694 doi: 10.1038/ncomms3694 (2013).